Electrically tunable nonlinear plasmonics in graphene nanoislands Nonlinear optical processes rely on the intrinsically weak interactions between photons enabled by their coupling with matter. Unfortunately, many applications in nonlinear optics are severely hindered by the small response of conventional materials. Metallic nanostructures partially alleviate this situation, as the large light enhancement associated with their localized plasmons amplifies their nonlinear response to record high levels. Graphene hosts long-lived, electrically tunable plasmons that also interact strongly with light. Here we show that the nonlinear polarizabilities of graphene nanoislands can be electrically tuned to surpass by several orders of magnitude those of metal nanoparticles of similar size. This extraordinary behaviour extends over the visible and near-infrared spectrum for islands consisting of hundreds of carbon atoms doped with moderate carrier densities. Our quantum-mechanical simulations of the plasmon-enhanced optical response of nanographene reveal this material as an ideal platform for the development of electrically tunable nonlinear optical nanodevices. The well established field of nonlinear photonics hosts a vast number of applications, including spatial and spectral control of laser light, all-optical signal processing, ultrafast switching and sensing [1] , [2] . Because the efficiencies of nonlinear optical processes are generally poor, considerable effort has been devoted towards seeking materials that can display nonlinear effects at low light intensities and ultrafast response times [2] , [3] , [4] . For this purpose, plasmonic nanostructures have been particularly attractive due to their ability to generate high local intensity enhancements through strong confinement of electromagnetic fields [3] , [5] , [6] , leading to second-harmonic polarizabilities as high as ~10 −27 esu (electrostatic units) per atom, as measured for noble metal nanoparticles [3] , and even beating the best molecular chromophores [3] , [7] , [8] . However, although localized plasmons can be customized through the size, shape and surrounding environment of the metal nanostructures [5] , they suffer from low lifetimes and lack post-fabrication tunability [9] . Doped graphene has recently attracted much attention as an alternative plasmonic material capable of sustaining electrically tunable optical excitations with long lifetimes [9] , [10] , [11] , [12] , [13] , [14] , [15] , [16] , [17] , [18] . The existence of gate-tunable plasmons in graphene has been confirmed by THz [13] , [14] and mid-infrared [15] , [16] spectroscopies, while optical near-field microscopy has been used to image them in real space [17] , [18] . Efforts to extend the plasmonic response of graphene to the visible and near-infrared regimes are currently underway [12] . In addition, graphene has been predicted to display intense nonlinearity due to its anharmonic charge–carrier dispersion relation [19] . Recent four-wave mixing [20] , Kerr effect [21] , and third-harmonic generation (THG) [22] experiments already confirm a large third-order response in this material in the undoped, plasmon-free state. Graphene plasmons could amplify this response further [23] , and even enable strong few-photon interactions in small islands [24] , [25] . Here we show that the nonlinear optical polarizabilities of small graphene nanoislands (<10 nm) exceed by several orders of magnitude those of noble metal nanoparticles with similar lateral size (but obviously of much greater volume), which are among the best nonlinear materials. Nonlocal and finite-size effects dominate the response of these structures [26] , [27] , which we model in a quantum-mechanical fashion. Specifically, we perform density-matrix simulations using a tight-binding description of the electronic states and following complementary time-domain and perturbative approaches (see details in Methods). Our results reveal unprecedented levels of nonlinearity when the graphene nanoislands are doped with only a few electrons. 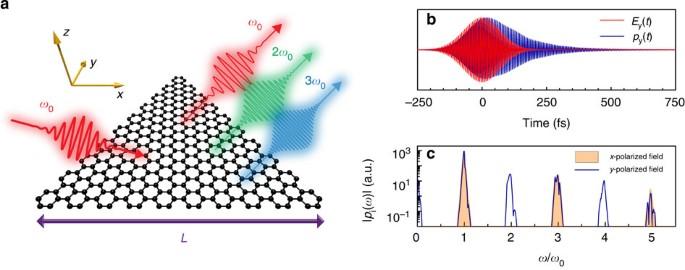Figure 1: Nonlinear response of nanographene. (a) Illustration of a doped graphene nanotriangle (armchair edges,N=330 carbon atoms,L=4.1 nm side length, doped withQ=2 additional charge carriers) under irradiation by a short light pulse (166 fs full width at half maximum (FWHM) duration, 1012W m−2peak intensity,ℏω0=0.68 eV central energy) tuned to one of the graphene plasmons. (b) Time variations of the incident electric field and the induced graphene dipole. (c) Harmonic analysis of the graphene dipole for polarizations along thexandydirections (see axes ina). Harmonic generation by an ultrashort pulse Figure 1 illustrates the optical nonlinearity of one of the armchair-edged triangular graphene nanoislands considered in this work, consisting of 330 carbon atoms, spanning a side length of 4.1 nm and doped with two additional charge carriers (2.3 × 10 13 cm −2 doping density, equivalent to 0.56 eV Fermi energy in extended graphene). Upon illumination with a light pulse of central energy ℏ ω 0 =0.68 eV, tuned to one of its plasmons, the island is capable of producing significant nonlinear polarization at multiple harmonics ( Fig. 1a ), including second-harmonic generation (SHG) and THG. The temporal evolution of the induced polarization ( Fig. 1b , blue) and its spectral decomposition (Fourier transform, Fig. 1c ) show the excitation of high harmonics using a relatively moderate pulse fluence 177 mJ m −2 (see Supplementary Fig. 1 for additional results obtained from various incident fluences). Although graphene is a centrosymmetric two-dimensional crystal, which ordinarily would prevent even-ordered nonlinear processes from occuring [1] , this symmetry can be broken by the finite size of the nanoisland. Notice that the mirror symmetry of the nanoisland along x results in the vanishing of even-harmonic generation when the incident light is polarized along that direction. Conversely, both odd and even harmonics are observed with a pulse polarized along the asymmetric y direction. Interestingly, the intensity of odd harmonics is independent of polarization direction because the nanoisland has threefold rotational symmetry. For the pulse polarized along the y direction, we also take special note of a static electric field formed in the graphene nanoisland due to optical rectification, as indicated by the polarization emerging at zero frequency in Fig. 1c . Figure 1: Nonlinear response of nanographene. ( a ) Illustration of a doped graphene nanotriangle (armchair edges, N =330 carbon atoms, L =4.1 nm side length, doped with Q =2 additional charge carriers) under irradiation by a short light pulse (166 fs full width at half maximum (FWHM) duration, 10 12 W m −2 peak intensity, ℏ ω 0 =0.68 eV central energy) tuned to one of the graphene plasmons. ( b ) Time variations of the incident electric field and the induced graphene dipole. ( c ) Harmonic analysis of the graphene dipole for polarizations along the x and y directions (see axes in a ). Full size image Electrically tunable nonlinear response For a quantitative analysis of the linear and nonlinear optical response of nanographene, we examine the incident-frequency dependence of the nonlinear polarizability in Fig. 2 . Both time-domain and perturbative approaches produce nearly identical results when the former is computed for low light intensities (see Methods). For simplicity, we concentrate on the same nanotriangle as in Fig. 1 , under different doping conditions, ranging from Q =0 to Q =6 additional charge carriers. In undoped graphene ( Q =0), the linear polarizability ( Fig. 2a ) is dominated by a single >1 eV plasmon in the spectral region under consideration, which, however, produces only negligible SHG ( Fig. 2b ) and THG ( Fig. 2c ). In contrast, when the island is doped, <1 eV plasmon features emerge ( Fig. 2a ), which move towards higher energies as Q is increased. These highly tunable, low-energy dipole plasmon modes are a result of the collective nature of the electronic excitations of the nanoisland, and do not coincide with any dominant electron–hole pair transitions [12] , [28] . Incidentally, zigzag edges are detrimental for the emergence of these plasmons and the resulting tunable nonlinear response (see Supplementary Figs 4 and 5 ). Importantly, intense features appear in the nonlinear spectra at incident photon energies tuned to the low-energy plasmons ( Fig. 2b,c ). These features exhibit multicomponent line profiles that indicate a complex interplay between the responses at the incident frequency and at multiples of that frequency. The nonlinear strengths follow a non-monotonic evolution with Q that we also attribute to that interplay (see below). For quantitative comparisons with bulk materials, we approximate the nonlinear susceptibilities χ (2) and χ (3) in doped nanographene by considering the polarizability per atom (denoted here as for the harmonic s ) and calculating , where n C =3.8 × 10 15 cm −2 is the areal density of carbon atoms in graphene and d gr ≃ 3.3 × 10 −8 cm is the effective thickness of a graphene layer (see right vertical axes in Fig. 2 ). For comparison, we note that the third-order susceptibility of extended graphene without the involvement of any plasmons has been measured via four-wave mixing experiments as | χ (3) |~10 −7 esu, exceeding the maximum value obtained for a 4-nm-thick gold film measured under the same experimental conditions [20] . In addition, THG measurements have yielded values | χ (3) |~10 −8 esu in graphene [22] . 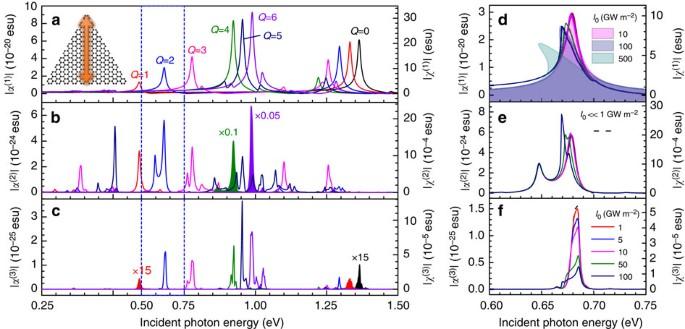Figure 2: Linear and nonlinear polarizability spectra. We study the nanotriangle ofFig. 1for external polarization perpendicular to one of the graphene sides, assuming different doping levels as indicated by the number of additional charge carriersQ. (a–c) Linear (a), second-harmonic (b) and third-harmonic (c) polarizabilities for low-intensity continuous illumination. (d–f) Same asa–ccalculated for various high intensitiesI0, and at frequencies near the lowest-energy dipole plasmon underQ=2 doping, as indicated by the vertical dashed blue lines spanninga–c. The filled curves inbandchave been multiplied by the factors indicated with text of the corresponding colour, while the filled curves indare obtained with a classical anharmonic oscillator model (see main text). Figure 2: Linear and nonlinear polarizability spectra. We study the nanotriangle of Fig. 1 for external polarization perpendicular to one of the graphene sides, assuming different doping levels as indicated by the number of additional charge carriers Q . ( a – c ) Linear ( a ), second-harmonic ( b ) and third-harmonic ( c ) polarizabilities for low-intensity continuous illumination. ( d – f ) Same as a – c calculated for various high intensities I 0 , and at frequencies near the lowest-energy dipole plasmon under Q =2 doping, as indicated by the vertical dashed blue lines spanning a – c . The filled curves in b and c have been multiplied by the factors indicated with text of the corresponding colour, while the filled curves in d are obtained with a classical anharmonic oscillator model (see main text). Full size image The linear and nonlinear spectral lineshapes display a dependence on light intensity that is clearly observable above ~1 GW m −2 , as shown through time-domain simulations in Fig. 2d–f , obtained from the Fourier transform of the induced dipole over an optical cycle after reaching a steady-state regime (see Methods). In particular, the third-order nonlinearity contributes to the polarization oscillating at the incident frequency ω through the Kerr effect [1] , the spectral details of which can be actually mimicked by a classical model, assuming that each electron of mass m e oscillates around its equilibrium position x =0 driven by the incident field and subjected to an anharmonic potential of resonance energy ℏ ω 0 =0.68 eV and nonlinear coefficient a . Using a fixed value a =−(4.7+0.3 i ) × 10 47 m −2 s −2 , this model reproduces the initial redshift with increasing intensity I 0 found in the calculated linear polarizability for I 0 =10 10 −10 11 W m −2 (see Fig. 2d and Methods), while it predicts optical bistability at even higher intensities ( I 0 =5 × 10 11 W m −2 ). The number of electrons involved in the observed resonances, as estimated from the f -sum rule [12] , [29] , is roughly proportional to the resonance frequency times the maximum polarizability, where the latter is given by the area of the symbols in the top panel of Fig. 3a . Although the largest islands studied here involve many electrons in each resonance according to this criterium, and thus, we can legitimately talk about plasmon resonances, it is interesting to note that the mode examined in Fig. 2d for the 330-atom triangle has an effective strength of only ~0.3 electrons. However, the energy of this mode is very different from those of individual dipole-active electron–hole pair excitations [28] , which emphasizes its many-body character. It is nonetheless surprising that nonlinear effects are observed at relatively moderate intensities (for example, 10 11 W m −2 ), for which the excited state still has a low population n p ~0.08, as estimated by equating the energy absorbed by the particle (that is, σ abs I 0 , where σ abs ≈(4 πω / c )Im{ α (1) } is the absorption cross-section) to the energy dissipated through plasmon decay (that is, n p ℏ ω p / τ , where ω p and τ are the mode frequency and decay time, respectively). 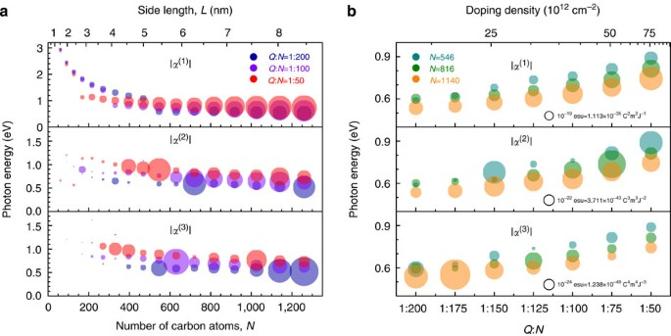Figure 3: Evolution of the nonlinear response with graphene size and doping level. We show linear and nonlinear peak polarizabilities (proportional to symbol areas, see empty-circle scales inb) at the dominant plasmon features of graphene armchair nanotriangles as a function of their size (a) and doping level (b) for selected doping levels and sizes, respectively. The vertical positions of the symbols indicate the resonant incident light energies. Figure 3: Evolution of the nonlinear response with graphene size and doping level. We show linear and nonlinear peak polarizabilities (proportional to symbol areas, see empty-circle scales in b ) at the dominant plasmon features of graphene armchair nanotriangles as a function of their size ( a ) and doping level ( b ) for selected doping levels and sizes, respectively. The vertical positions of the symbols indicate the resonant incident light energies. Full size image Mapping the nonlinearity in doped graphene nanoislands We present in Fig. 3 an overview of the dependence of the maximum first-, second-, and third-harmonic polarizabilities on island size and doping (see also Supplementary Fig. 2 for the polarizabilities normalized to the number of atoms). The linear polarizabilities increase monotonically with size and doping, while the plasmon energies scale roughly as ~ Q 1/4 / N 1/2 , in a way that is consistent with a local classical description of the optical response [12] . With fixed doping densities, the maximum linear polarizability is found among the higher-energy plasmon modes for smaller islands, as illustrated in Fig. 2a for low doping. As the nanoisland size increases, and with it the doping level, the lower-energy modes eventually become dominant. In contrast, the nonlinear polarizabilities exhibit a non-monotonic evolution with both Q and N , which we again attribute to the presence of resonances at both the fundamental and the harmonic frequencies. When normalized per carbon atom, the THG susceptibilities take extraordinarily large values | χ (3) |~10 −6 –10 −4 esu (see Supplementary Fig. 2 and below). A mechanism of double plasmonic enhancement is illustrated in Fig. 4 , showing anomalously large nonlinear polarizabilities when a plasmon exists at a multiple of the fundamental frequency, which is in turn tuned to another plasmon. This phenomenon has been recently invoked to predict nonlinearities in graphene islands at the single-photon level [25] . For SHG, Fig. 4a shows this effect taking place for an island consisting of N =168 atoms. Similarly, Fig. 4b shows large THG with N =270. The non-monotonic evolution of the nonlinear polarizabilities with size and doping noted in Figs 2 and 3 are also due to this type of double-resonance effect. For a fixed geometry, the double-enhancement phenomenon should be attainable by varying the doping charge density: consider, for example, the highly tunable, low-energy dipole plasmon mode of Fig. 2a , which evolves with doping, eventually converging to the less-tunable, higher-energy mode, so that at some point before converging the two modes satisfy the required 1:2 energy ratio. This phenomenon should also occur in imperfect nanoislands with a predominance of armchair edges, although higher levels of doping could be necessary (see Supplementary Fig. 6 ). 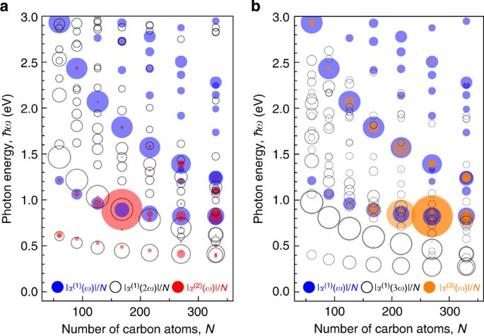Figure 4: Doubly resonant SHG and THG. Local maxima in the polarizability spectra, normalized to the number of carbon atoms, are shown for various nanoislands with a fixed doping carrier densityN/Q=100. The filled symbols show the linear and nonlinear polarizabilities as functions of the fundamental incident photon frequency, while the empty symbols show the linear polarizability at the indicated harmonic frequency (see legends). Large SHG (a) and THG (b) is observed for nanoislands that support plasmons at both the fundamental frequency and twice or three times that frequency, respectively. The polarizability is proportional to the area of the symbols. Figure 4: Doubly resonant SHG and THG. Local maxima in the polarizability spectra, normalized to the number of carbon atoms, are shown for various nanoislands with a fixed doping carrier density N / Q =100. The filled symbols show the linear and nonlinear polarizabilities as functions of the fundamental incident photon frequency, while the empty symbols show the linear polarizability at the indicated harmonic frequency (see legends). Large SHG ( a ) and THG ( b ) is observed for nanoislands that support plasmons at both the fundamental frequency and twice or three times that frequency, respectively. The polarizability is proportional to the area of the symbols. 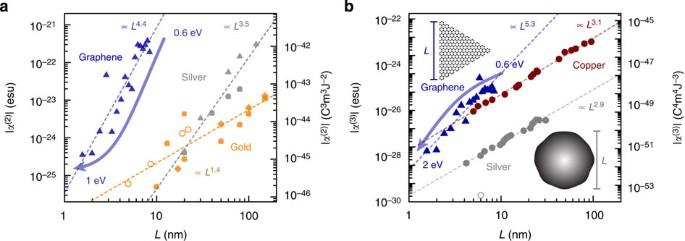Figure 5: Second- and third-harmonic responses of nanographene compared with noble metal nanoparticles. We show the nonlinear polarizabilities of graphene nanotriangles (solid blue triangles) as a function of their side lengthLat a fixed doping of one electron per 100 carbon atoms, compared with measured values of noble metal nanoparticles (MNPs) of the same maximum length. Inawe show second-harmonic data for roughly spherical gold and silver MNPs measured at fundamental wavelengths of 800 and 780 nm, respectively (solid circles)7,8; roughly spherical gold MNPs measured at a fundamental wavelength of 1,064 nm (open circles)30; gold decahedra measured at a fundamental wavelength of 790 nm (solid diamonds)31; and silver triangles measured at a fundamental wavelength of 1,064 nm (solid triangles)32. Inbwe show degenerate four-wave mixing data for roughly spherical silver and copper MNPs measured at wavelengths of ~420 and ~570 nm, respectively (solid circles)33, as well as THG data for silver MNPs measured at a fundamental wavelength of 1,230 nm (open circle at the bottom)34. Dashed lines are added to indicate the approximate scaling withLaccording to experimental observations. The calculated graphene polarizabilities correspond to incident light energies as indicated along the curved arrows. Full size image Comparison to noble metal nanoparticles Figure 5a shows that the SHG polarizabilities predicted for nanographene exceed by three orders of magnitude the optimal values measured for noble metal nanoparticles of similar lateral size. For a comprehensive comparison of SHG with noble metals, we present data from experiments performed on various nanoparticle morphologies, including highly asymmetric structures, as well as for different excitation frequencies [8] , [30] , [31] , [32] . The comparison per unit volume is even more favourable to graphene, as it is an atomically thin structure, in contrast to the three-dimensional nanoparticles. The third-order polarizability in graphene is also above that measured for copper and silver [33] , [34] ( Fig. 5b ), and more so when considering that these measurements refer to fully degenerate four-wave mixing experiments, which tend to yield significantly higher values than those obtained when looking at THG or non-degenerate four-wave mixing [35] . Although larger graphene islands present a computational challenge beyond our current computational capabilities, the pace at which their nonlinear polarizabilities increase with size should be faster than that of noble metals, as expected from the extrapolation of the dashed lines in Fig. 5 . It should be noted that this occurs at plasmon energies that eventually evolve towards the mid-infrared (see Fig. 3a ), whereas the size range here explored yields tunable visible and mid-infrared excitations. Figure 5: Second- and third-harmonic responses of nanographene compared with noble metal nanoparticles. We show the nonlinear polarizabilities of graphene nanotriangles (solid blue triangles) as a function of their side length L at a fixed doping of one electron per 100 carbon atoms, compared with measured values of noble metal nanoparticles (MNPs) of the same maximum length. In a we show second-harmonic data for roughly spherical gold and silver MNPs measured at fundamental wavelengths of 800 and 780 nm, respectively (solid circles) [7] , [8] ; roughly spherical gold MNPs measured at a fundamental wavelength of 1,064 nm (open circles) [30] ; gold decahedra measured at a fundamental wavelength of 790 nm (solid diamonds) [31] ; and silver triangles measured at a fundamental wavelength of 1,064 nm (solid triangles) [32] . In b we show degenerate four-wave mixing data for roughly spherical silver and copper MNPs measured at wavelengths of ~420 and ~570 nm, respectively (solid circles) [33] , as well as THG data for silver MNPs measured at a fundamental wavelength of 1,230 nm (open circle at the bottom) [34] . Dashed lines are added to indicate the approximate scaling with L according to experimental observations. The calculated graphene polarizabilities correspond to incident light energies as indicated along the curved arrows. Full size image The magnitudes of the second- and third-order nonlinear polarizabilities of doped graphene nanoislands predicted by our simulations are several orders of magnitude higher than those reported for noble metal nanoparticles with comparable lateral sizes. We note that the polarizabilities of noble metals measured experimentally may be less than those that could be obtained from rigorous theoretical calculations, and thus it would be prudent to compare the latter for noble metal nanoparticles, particularly for geometries that optimize signals at both the fundamental and harmonic frequencies (that is, via double plasmon resonance at both frequencies). Nevertheless, the extraordinary SHG and THG reported above warrants further exploration of nonlinear optical phenomena in doped nanographene. Other morphologies apart from nanotriangles should yield similar high levels of nonlinear response, particularly when their edges are predominantly armchair. Graphene nanoislands with sizes comparable to those considered here have already been fabricated using various methods [36] , [37] , [38] , although they lack precise control over size and shape, which limits their applicability to nonlinear photonic technologies. Alternatively, a bottom-up approach based upon chemical self-asembly of molecular precursors provides better degree of control over the sizes and edge configurations [39] , [40] , [41] . In practical devices, electrical doping can be introduced in the nanoislands through a transparent substrate [42] , or by placing them close to a contact, from which electrons can be tunnelled. Arrayed nanoislands can transform a substantial fraction of the incident light energy into nonlinear harmonics (see Supplementary Fig. 7 ). Our results indicate that a relatively small amount of charge transferred to a graphene nanoisland can facilitate a marked increase in the magnitude of the nonlinear polarizability. This suggests the use of graphene nanoislands for the development of nanometre-sized optoelectronic switches and modulators, as well as for the detection of minute amounts of analytes through their charge transfer to the graphene. Introduction We investigate the linear and nonlinear optical response of doped graphene nanoislands, with emphasis on enhanced nonlinearities arising when the involved optical frequencies are tuned to the graphene plasmons. The latter correspond to light wavelengths that are much larger than the size of the islands [10] , and therefore, we characterize their optical response in the electrostatic limit, so they contribute to the far field with their induced dipole moment p . In our numerical simulations, we consider light incident along the direction normal to the carbon plane, which we take as . As we are interested in the enhanced optical response due to plasmons, armchair-edged nanoislands are preferred because they support intense and highly tunable modes, whereas zigzag-edged islands host near-zero-energy electronic states that are detrimental to the strength and tunability of optical excitations [28] , particularly when the plasmon energy is above the Fermi level [12] (see Supplementary Fig. 4 ). We concentrate on armchair nanotriangles lying on the x – y plane and oriented as illustrated in Fig. 1a of the main paper. However, the methods that we introduce below can be directly applied to arbitrarily shaped nanographene. We use a simple tight-binding representation for the low-energy electronic states of graphene, with one perpendicularly oriented p orbital per carbon atom [43] , [44] (see below). This model implicitly assumes that, for low excitation energies (<3 eV), the localized electrons in the σ band and the remaining in-plane p orbitals do not contribute significantly to the optical response other than by introducing a rather homogenous charge screening through their polarization, which slightly redshifts plasmon energies. These effects are not qualitatively changing the optical response, as compared with time-dependent density functional theory [27] , so we neglect them for simplicity. It should also be noted that excitonic effects can play a relevant role at the highest energies under consideration [45] , particularly for relatively small nanoislands in the absence of any doping [46] , although we do not attempt to describe these effects accurately. Density-matrix approach to the nonlinear optical response We model the optical response using a single-particle density-matrix approach, assuming that only π-band valence electrons are contributing and expanding them in a basis set formed by the 2p carbon orbitals oriented perpendicular to the graphene plane, with one spin-degenerate state | l › per atomic site R l =( x l , y l ). We adopt a tight-binding description [43] , [44] in which the unperturbed system is characterized by a Hamiltonian H TB of matrix elements ‹ l | H TB | l ′›=− hδ ‹ l , l ′› , where h =2.8 eV is the hopping energy, while δ ‹ l , l ′› is 1 if l and l ′ are nearest-neighbour carbon sites and 0 otherwise. Upon diagonalization of H TB , we obtain single-electron states of energies ℏ ε j that can be expressed as where the expansion coefficients a jl are real and give the amplitude of orbitals | l › in states j . These states are orthonormal (∑ l a jl a j ′ l = δ jj ′ ) and form a complete set (∑ j a jl a jl ′ = δ ll ′ ). In what follows, we use indices l to label carbon sites and j for single-electron states. We describe the electronic state of a graphene nanostructure through its single-particle density matrix ρ where are time-dependent matrix elements in the site (state) representation. We can move between these two representations using the relations and , involving the a jl coefficients defined in equation (1). Plasmon dynamics are then studied by solving the equation of motion [47] where is the system Hamiltonian, φ is the total potential acting on the graphene island and ρ 0 is the equilibrium density matrix at time t =−∞ (that is, before any interaction with external fields), to which the system relaxes at a rate τ −1 . The factor of 1/2 in the dissipation term of equation (2) accounts for the fact that we are relaxing to the ground state instead of the local thermal equilibrium state [48] . We construct from the incoherent filling of electron states according to the Fermi–Dirac-distribution occupation numbers f j [47] . Although this relaxation approximation is unable to conserve local electron density [48] , it should provide an accurate description for optical field components oscillating at frequencies ω ≫ τ −1 . This is the case of plasmons in high-quality doped graphene, for which we assume a realistic phenomenological inelastic relaxation rate ℏ τ −1 =10 meV throughout this work, unless otherwise stated (see Supplementary Fig. 3 ). It should be noted that the nonlinearity arises from the induced part of the potential, which produces a quadratic dependence on ρ on the right-hand side of equation (2). We obtain linear and nonlinear nanographene polarizabilities by numerically solving equation (2) using either time-domain or perturbative methods, as outlined in the following sections. In particular, results presented in Figs 1 and 2d–f and in Supplementary Figs 1 and 5 are obtained from time-domain simulations, while the results of Figs 2a–c and 3 , 4 , 5 and Supplementary Figs 2–4, 6 and 7 are calculated using the perturbative approach. Time-domain approach Direct numerical integration of the equation of motion (2) constitutes an intuitive method of solution, for which it is convenient to express it in the basis set of carbon site orbitals | l › as The elements of the Hamiltonian (see equation (3)) are Here, the total potential φ is diagonal in the site representation and results from the sum of the external potential where E ( t ) is the incident electric field, assumed to be uniform along the island, and the self-consistent induced potential, which we model in the Hartree approximation as [47] after correcting for homogeneous doping in the graphene nanoisland [49] . Here, is the induced charge at site l ′, ε ll ′ gives the spatial dependence of the Coulomb interaction between electrons in orbitals | l › and | l ′› [26] , and the factor of 2 accounts for electron spin. The time-dependent elements ρ ll ′ are calculated by numerically integrating equation (4) to yield the induced dipole moment We use this approach to study the response to high-fluence Gaussian light pulses (see Fig. 1 in the main text and Supplementary Fig. 1 ). In addition, we are interested in computing SHG and THG upon continuous-wave (CW) illumination. Accordingly, we write the incident field as where is the polarization vector, which we take for simplicity along a high-symmetry direction of the system, so that the induced dipole is also along (this is the case for polarization either parallel or perpendicular to one of the sides of an equilateral triangular island). For moderate light intensities, the leading contribution to the dipole oscillating at the s th harmonic is defined as where α ( s ) is the s order polarizability. We calculate the latter by separating it from all other constituent terms in the induced dipole p ( t ) upon Fourier transformation of a single optical cycle. More precisely, from the above definition of p ( s ) ( t ) it follows that where we assume the system to have evolved to a steady state at a time t 1 ≫ τ after starting the simulation. We use this procedure to compute the frequency-dependent linear and nonlinear polarizabilities represented in Fig. 2d–f of the main paper and in Supplementary Fig. 5 . Perturbative approach An iterative solution of equation (2) is possible under CW illumination. This is facilitated by writing it in the state representation as where we have used H TB | j ›= ℏ ε j | j ›, and the interaction potential term has been transformed using the coefficients a jl of equation (1). We then expand the density matrix as where n =1, 2, 3, ... labels the perturbation order (that is, terms proportional to ( E 0 ) n , see equation (6)), while s indicates the harmonic. We use the property to reduce the computation time and storage demand roughly by a factor of 2. To 0th order in E 0 , equation (7) is trivially satisfied with ρ ns = δ s ,0 ρ 0 . The external potential contributes to first order ( n =1) with s =±1 components only. We obtain the solution at higher orders by inserting equation (8) into equation (7) and identifying terms with the same e −i sωt dependence on both sides of the equation. Clearly, we have | s |≤ n by construction. At order n ≥1, we find where while is the contribution to the harmonic s of the total potential at order n . In equation (9), the first term on the right-hand side has a linear dependence on ρ ns through the induced part of φ ns (that is, the sum in equation (11)), whereas we have separated the dependence on lower perturbation orders in . At each order n we are thus dealing with a self-consistent system in φ ns , which we handle in a way similar to the random-phase approximation formalism in the linear response theory [47] . We proceed by first using the identity in the sum of equation (9), and then moving from state to site representation to obtain the diagonal density-matrix elements as where is the noninteracting random-phase approximation susceptibility at frequency sω . In summary, each new iteration order n is computed from the results of previous orders as follows: (1) We first calculate using equation (10). (2) We then combine equations (11) and (12) to find a self-consistent equation for , which reduces in matrix form to using site labels l as matrix indices and having defined (3) We use the calculated values of and to obtain using equation (12), and from here the induced charge at site l at order n associated with harmonic s as . Incidentally, we can also calculate the full density-matrix using equation (9). (4) Finally, the polarizability of order s is calculated from upon iteration of this procedure up to order n = s . Nonlinear polarizability units In the literature, the nonlinear polarizabilities α (2) and α (3) are commonly reported in Gaussian electrostatic units (esu) [1] , [50] , with length in cm and charge in statcoulomb (1 statC=4 πc 0 C, where c 0 =2,997,924,580 is the speed of light expressed in m s −1 ), whereas many theoretical studies use atomic units (a.u., with e = ℏ = m e =1). The conversion factors between esu, SI and a.u. are given in Table 1 . Table 1 Polarizability conversion factors. Full size table Throughout this work we adopt the common convention of referring to the esu units of α (1) (cm 3 ), α (2) (cm 5 statC −1 ) and α (3) (cm 7 statC −2 ) simply as ‘esu’ [50] . For completeness, in Fig. 5 we compare our simulated nonlinear polarizabilities α (2) and α (3) with previously reported measurements for noble metal nanoparticles, and offer both esu and SI values, as obtained by using the noted table. In particular, we show the reported experimental values of | α (2) | acquired through hyper-Rayleigh scattering of various types of gold and silver nanoparticles in aqueous suspensions [7] , [8] , [30] , [31] , [32] . In addition, we show values of the reported third-order susceptibility | χ (3) | obtained from degenerate four-wave mixing measurements of glasses doped with silver and copper nanoparticles [33] and from THG measurements of dispersed silver colloids on quartz [34] , converted into | α (3) | upon multiplication by the particle volume. Anharmonic oscillator model The intensity dependence of the first-harmonic polarizability can be qualitatively described by a classical model for damped and optically driven particles of mass m e subjected to an effective anharmonic potential [51] , [52] . The equation of motion for such an oscillator can be written as where f quantifies the coupling strength to the driving electric field E ( t )= E 0 e −i ωt +c.c., while is the anharmonic potential, characterized by a resonance frequency ω 0 and a nonlinear coefficient a . The solution for the particle position x ( t ) can be expressed in harmonics of the driving field as If we neglect terms of order s >1 in the above expansion, equation (15) leads to for the first-harmonic amplitude x (1) . The cubic equation (16) can be used to explain the results obtained from our time-domain simulations for the linear polarizability of nanographene under intense CW illumination. In Fig. 2d of the main paper, we successfully fit α (1) =− ex (1) / E 0 to this model for one of the islands by taking ℏ ω 0 =0.68 eV, f =1.77 and a =−(4.7+0.3 i ) × 10 47 m −2 s −2 . It should be noted that the anharmonic oscillator model described here must be considered as a phenomenological tool, used simply to qualitatively illustrate the magnitude of the nonlinear shift observed in the linear spectra for illumination by intense, CW fields. Effect of the relaxation rate The large linear and nonlinear polarizabilities found in the graphene nanoislands depend strongly on the choice of the plasmon relaxation rate τ −1 . Throughout this work, unless otherwise specified, we take ℏ τ −1 =10 meV, which is comparable to the values estimated from d.c. impurity-limited mobilities in high-quality graphene [53] , [54] , [55] and similar to values reported for graphene used in actual plasmonic studies [42] . This is a conservative choice, because chemical synthesis of finite-sized nanoislands should enable fabrication of nanographene with fewer defects and less disorder. Arguably, graphene phonons may also contribute to losses via phonon–plasmon coupling decay channels, in particular for optical phonons near ~0.2 eV (ref. 55 ). These modes are essentially connected with the stretching oscillations of C–C bonds, so they are very localized and give rise to relatively dispersionless bands. Therefore, their contribution to inelastic attenuation acts locally and we expect them to behave in a similar way as in extended graphene even in small nanoislands. Nanoisland arrays The experimental realization of SHG and THG from graphene nanoislands could benefit from using samples containing large numbers of nanoislands. We estimate here the nonlinear signal intensity resulting from an array of nanotriangles illuminated by a light plane wave. For simplicity, we consider a square array under normal incidence conditions. From the response of a dipole array, the linear reflected electric field is given by the expression [56] where G ( ω )≈4.52/ a 3 + i [ S ( ω )−2 ω 3 /3 c 3 ] is a lattice sum that accounts for the dipole–dipole interactions between nanoislands, a is the period of the array and S ( ω )=2 πω / ca 2 , assuming ωa / c ≪ 1. Now, we extend this approach to describe higher harmonics in terms of the nonlinear polarizabilities. A straightforward generalization of the methods in ref. 56 permits writing the intensity of the s harmonic normalized to the incident intensity I 0 as We show in Supplementary Fig. 7 the power emitted towards one side of an array at frequencies sω for a period a =10 nm and islands like those of Fig. 2 of the main paper, using the nonlinear polarizabilities reported in that figure. For example, a peak intensity of 1 GW m −2 (100 GW m −2 ) will produce 1.3 W m −2 (13 kW m −2 ) and 0.29 W m −2 (0.29 MW m −2 ) via SHG and THG, respectively, when the nanoislands are doped with Q =2 (see Supplementary Fig. 7b ). How to cite this article : Cox, J. D. and García de Abajo, F. J. Electrically tunable nonlinear plasmonics in graphene nanoislands. Nat. Commun. 5:5725 doi: 10.1038/ncomms6725 (2014).